Photon extrabunching in ultrabright twin beams measured by two-photon counting in a semiconductor For many years twin beams originating from parametric down-converted light beams have aroused great interest and attention in the photonics community. One particular aspect of the twin beams is their peculiar intensity correlation functions, which are related to the coincidence rate of photon pairs. Here we take advantage of the huge bandwidth offered by two-photon absorption in a semiconductor to quantitatively determine correlation functions of twin beams generated by spontaneous parametric down-conversion. Compared with classical incoherent sources, photon extrabunching is unambiguously and precisely measured, originating from exact coincidence between down-converted pairs of photons, travelling in unison. These results strongly establish that two-photon counting in semiconductors is a powerful tool for the absolute measurement of light beam photon correlations at ultrashort timescales. The study and use of spontaneous parametric down-conversion (SPDC), a specific quantum effect with no classical equivalent [1] , [2] , constitutes an extensive research field at the heart of quantum optics, as a test bench of quantum effects, and also with a perspective of several promising applications such as quantum cryptography [3] , [4] and ghost imaging [5] . An irreplaceable tool for testing quantum correlation properties of light is the measurement of second-order correlation function ( g (2) ), expressed as: where Ê (+) ( t ) and Ê (−) ( t ) are the complex electric field operator and its hermitian conjugate, respectively, whereas 〈 〉 stands for quantum expectation [6] . g (2) ( τ ) is linked to the conditional probability of one photon arriving at time t + τ , knowing that another one previously arrived at time t (ref. 7 ). A popular g (2) measurement technique is the historical Hanbury–Brown and Twiss interferometer [8] , with further refinements such as refs 9 , 10 , 11 , 12 . More recently, Grosse et al . [13] devised an experiment coupling a Hanbury–Brown and Twiss interferometer with a homodyne detection set up. These authors were able to determine g (2) (0)≈3 for displaced thermal states but in the few tens of μs timescale. Indeed, the Hanbury–Brown and Twiss technique does not allow to measure g (2) ( τ ) at very short timescales because of the limited response time of the detectors [14] . Such a time resolution (nanosecond at best) cannot unravel the whole dynamics of SPDC twin beams. Measurement of the correlation function g (2) of a light pulse was also recently demonstrated by use of an alternative technique based on streak-camera detection [15] , [16] . However, the picosecond time resolution of this later technique is still too long to capture the dynamics of photon correlations within broadband SPDC twin beams. Except for two-photon interferences in the Hong–Ou–Mandel experiment [17] , which is limited to the detection of isolated biphotons, 'ultrafast' g (2) measurement techniques are based on the detection of photons or electrons produced by nearly instantaneous non-linear interactions. These techniques have been initially developed for ultrashort pulse duration measurement [18] , [19] , [20] , [21] . Most of them combine an interferometer and sum frequency generation as demonstrated by Abram et al . [22] , who carried out the first degenerate twin-beam autocorrelation measurement by using a modified Mach–Zehnder interferometer with a few tens of femtosecond resolution. Owing to improvements in crystal non-linearities and twin-beam dispersion compensation, the sensitivity of this up-conversion experiment was greatly improved by authors such as Dayan et al . [23] , O'Donnell et al . [24] or Sensarn et al . [25] , reaching the corpuscular regime where pairs are separate in time (that is, less than one photon per mode). A more recent technique for the study of the correlation properties of twin beams is based on two-photon absorption (TPA) in atoms. Georgiades et al . [26] , followed by Dayan et al . [27] , unravelled the peculiar behaviour of biphotons on TPA in caesium and rubidium atoms, such as a linear dependence of TPA on biphoton beam intensity. Striking effects regarding the correlation properties of twin beams were predicted in the 1970s such as additional g (2) ( τ ) contributions because of twin photons [7] , [28] . However, neither the atomic resonance TPA technique nor the sum frequency generation scheme allows to quantify this latter effect. Indeed these methods involve conservation properties (energy for the first one, plus momentum conservation for the second), which prevent uncorrelated pairs to be detected. It is thus impossible to rate correlated pairs relative to uncorrelated ones. In this paper, following previous g (2) experiments on broadband sources [29] , [30] , we use two-photon counting (TPC) in a semiconductor detector to measure g (2) for broadband SPDC sources at the femtosecond timescale. We show and characterize an unambiguous extrabunching effect with this SPDC source (that is, g (2) (0)≥3) compared with a classical chaotic source (that is, g (2) (0)=2) occurring at the 100 fs scale, which highlights the peculiar correlation properties of twin beams. This quantitative measurement of the extrabunching effect is enabled by the unique capability of our setup to distinguish real twin pairs and accidental coincidences. TPC in semiconductors TPC in semiconductors is very well adapted to study broadband and non-degenerate twin beams. Indeed, as TPA transition rates [31] are directly related to the expectation value of three different two-photon combinations enable a TPC event in a semiconductor ( Fig. 1a ). Two of them occur at degenerate wavelengths, that is, 'signal+signal'−TPC of energy or 'idler+idler'−TPC of energy and one at non-degenerate wavelengths, that is, 'signal+idler'−TPC of energy Next, as the lifetime of a virtual state held by an electron during the transition from a valence to conduction band state is very short, in the order of few femtoseconds [30] , TPC intrinsically fits for ultrashort time photon correlation study. Finally, recent progress in detector technology (such as very low dark counts) allows low-intensity continuous wave (CW) fields to be studied (that is, in the low 100 nW) [29] , [32] . Different intensity correlation functions are involved in these TPC processes, which are proportional to the generalized second-order correlation functions [7] : where ' k ' and ' l ' can stand for signal (' s ') or idler (' i '), Î k stands for the intensity operator and :: means normal ordering. Note that if the two beams are uncorrelated. Both degenerate TPC events are linked to self-signal and self-idler autocorrelation functions, and respectively, whereas non-degenerate TPC event enables to measure photon cross-correlation between signal and idler photon ( Fig. 1b ). We shall see below how our experimental setup independently determines these two different types of contributions (self and cross) to the TPC signal. 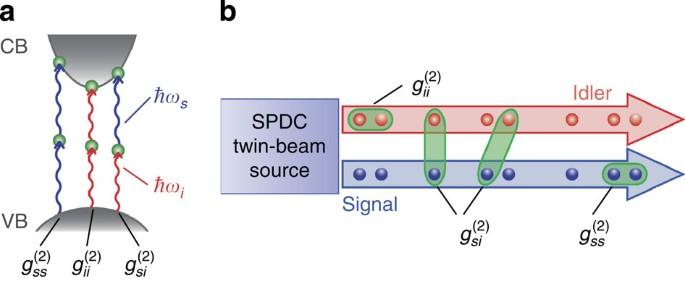Figure 1: Principles of correlation measurement of twin beams by TPC. (a) Transition of an electron by TPA from valence band (VB) states to conduction band (CB) states via a virtual state in direct-gap semiconductors is possible by three kinds of two-photon combinations: absorption of two signal (blue) photons, absorption of two idler (red) photons and/or absorption of one idler plus one signal photon. (b) Photon correlations of twin beams originate from idler photon correlationsignal photon correlationand correlation between signal and idler photonsThe vertical greenarrow symbolizes exact coincidence, whereas the oblique one stands for accidental ones. Figure 1: Principles of correlation measurement of twin beams by TPC. ( a ) Transition of an electron by TPA from valence band (VB) states to conduction band (CB) states via a virtual state in direct-gap semiconductors is possible by three kinds of two-photon combinations: absorption of two signal (blue) photons, absorption of two idler (red) photons and/or absorption of one idler plus one signal photon. ( b ) Photon correlations of twin beams originate from idler photon correlation signal photon correlation and correlation between signal and idler photons The vertical green arrow symbolizes exact coincidence, whereas the oblique one stands for accidental ones. 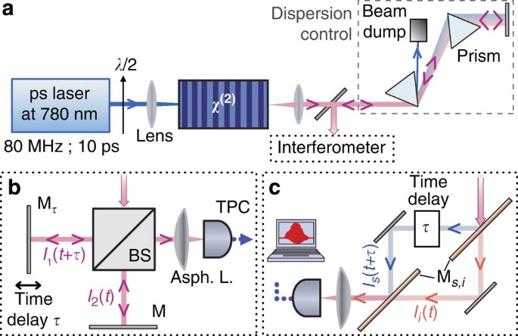Figure 2: Experimental setups. (a) The source is based on a non-linear crystal (χ(2)) pumped at 780 nm by a mode-locked Ti:sapphire laser delivering 10 ps pulses at 80-MHz repetition rate. The dispersion of the twin beams is compensated by a backward and forward propagation in a SF14 glass prism pair. The collimated beam then passes through the Michelson or modified Mach–Zehnder interferometer before being focused by a 26-mm aspheric lens (Asph. L) on a two-photon counter (TPC). Estimated focal spot on the detector is 5 μm. (b) The Michelson interferometer consists of two arms that are common for both signal and idler: BS is a 50/50 beam splitter, M and Mτare golden mirrors and the time delayτis adjusted by translating Mτ. (c) The modified Mach–Zehnder interferometer consists of two separate paths for signal and idler, which are split towards the two individual paths by a dichroic mirror (Ms,i) reflecting signal and transmitting idler wavelength. The time delayτis explored on the signal path. Full size image Photon correlation measurement setups Our experiment is presented in Figure 2a : the twin-beam source is based on a non-linear crystal, a type-0 35-mm-long periodically poled lithium niobate crystal, pumped at 780 nm by a mode-locked Ti:sapphire laser delivering 10 ps pulses at 80-MHz repetition rate. The collimated parametric beam of 50 μW mean power goes through a SF14 Brewster prism pair spaced by 73 mm and back to compensate for the chirp accumulated in all dispersive media of the setup. As only the exact coincidences originating from twin photons pairs are altered by chromatic dispersion [23] , [24] , [30] , adjusting compensation allows us to tune our source from highly correlated twin beams to two independent beams of the same spectrum. In addition, the prism pair efficiently filters out the pump radiation. The peak photon flux Φ max is 1.2×10 18 photons s −1 , that is, 4.9×10 6 photons per pulse. Given the approximate signal or idler beam bandwidth Δ in the few tens of THz, there are thus far more than one photon per mode ( Φ max /Δ ≫ 1) (ref. 23 ). These ultrabright twin beams are then sent through an interferometer and focused on a GaAs two-photon counter [29] . Figure 2: Experimental setups. ( a ) The source is based on a non-linear crystal ( χ (2) ) pumped at 780 nm by a mode-locked Ti:sapphire laser delivering 10 ps pulses at 80-MHz repetition rate. The dispersion of the twin beams is compensated by a backward and forward propagation in a SF14 glass prism pair. The collimated beam then passes through the Michelson or modified Mach–Zehnder interferometer before being focused by a 26-mm aspheric lens (Asph. L) on a two-photon counter (TPC). Estimated focal spot on the detector is 5 μm. ( b ) The Michelson interferometer consists of two arms that are common for both signal and idler: BS is a 50/50 beam splitter, M and M τ are golden mirrors and the time delay τ is adjusted by translating M τ . ( c ) The modified Mach–Zehnder interferometer consists of two separate paths for signal and idler, which are split towards the two individual paths by a dichroic mirror (M s , i ) reflecting signal and transmitting idler wavelength. The time delay τ is explored on the signal path. Full size image Two setups are used to evaluate the twin-beam correlation properties. The first one is a standard Michelson interferometric apparatus ( Fig. 2b ), where no distinction is made between signal and idler beams. The autocorrelation function g (2) ( τ ) of the whole twin-beam field, measured by this setup is easily expressed as: where Note that, assuming the signal and idler fields are chaotic sources when separately measured [30] , [33] , [34] , [35] (that is, this expression simplifies at zero delay as: In this latter expression, we have introduced the extrabunching parameter defined by to highlight how cross-correlations between beams may lead to an enhancement of the g (2) value compared with uncorrelated sources [7] . The second setup is a modified Mach–Zehnder interferometer ( Fig. 2c ), where the signal and idler beams are split upon two different paths by a dichroic mirror and recombined on a second one, thus avoiding any first-order interference effect [25] . Obviously, this second setup can be used only far from degeneracy. 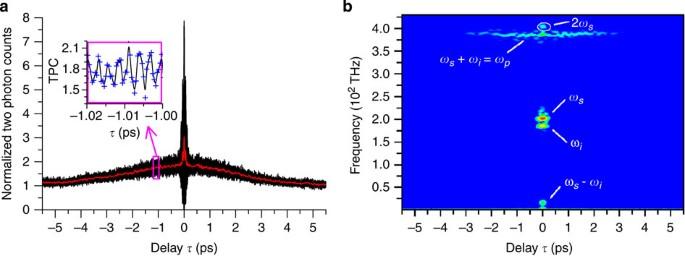Figure 3: TPC interferogram of non-degenerate twin beams using the Michelson setup. (a) TPC interferogram as a function of the delayτin the Michelson setup ofFigure 2b(black line) and low-pass filtered (red line). The left inset shows a zoomed part of the broad shoulders seen on main graphic (same units). (b) Time–frequency analysis of the TPC interferogram shown in (a). This setup measures the quantum expectation of the intensity of the twin-beam field, that is, leads directly to the intensity cross-correlation function Photon extrabunching in twin beams Figure 3a shows a typical TPC interferogram, TPC( τ ), carried out on the whole non-degenerate twin-beam pulse by use of the Michelson apparatus. The strong oscillations observed on this interferogram are reminiscent of the phase interference, whereas their contrast is linked to the optical non-linearities involved in this experiment [30] , [36] . Figure 3b shows a spectrogram of TPC( τ ) [37] , that is, a plot of the frequency components of TPC( τ ) as a function of the delay τ . One observes frequency components centred, respectively, at ω s =201 THz ( ∼ 1.49 μm) and ω i =184 THz ( ∼ 1.63 μm), which is in compliance with the signal and idler central frequencies measured experimentally. As demonstrated by the time width of the spots at signal and idler frequencies, their individual coherence times τ c are short compared with the pulse duration. This property allows us to conveniently use a continuous wave approach in our quantum and semiclassical modelling. An interesting feature of the spectrogram is the clear observation of the ω s + ω i = ω p frequency at 385 THz ( ∼ 780 nm) during almost the whole duration of twin-beam pulse. As neither signal nor idler frequencies are present at such a long delay, this oscillation reveals the already demonstrated two-photon interference effect originating from the coherence of the twin-beam field [9] , [10] , [38] . Figure 3: TPC interferogram of non-degenerate twin beams using the Michelson setup. ( a ) TPC interferogram as a function of the delay τ in the Michelson setup of Figure 2b (black line) and low-pass filtered (red line). The left inset shows a zoomed part of the broad shoulders seen on main graphic (same units). ( b ) Time–frequency analysis of the TPC interferogram shown in ( a ). Full size image The g (2) ( τ ) spectrum is extracted from the raw interferogram TPC( τ ) in the following way: The high-frequency parts are filtered out, leaving the low-frequency parts (that is, ω s − ω i and below), named TPC LF ( τ ) [30] (see red curve on Fig. 3 ). The interferogram TPC LF (τ) is normalized by TPC( τ ≫ τ c ) counts at long delay [36] . This possibility to have access to the uncorrelated part of the spectrum is thus primordial, as it enables us to obtain the absolute value of the function g (2) ( τ ) (see Methods). 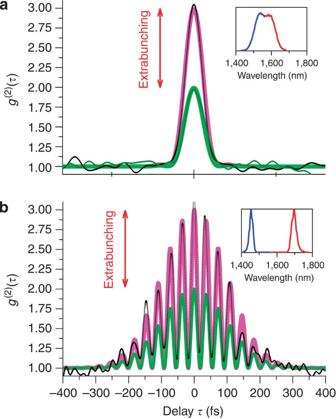Figure 4: Quantitative measurements of extrabunching. g(2)(τ) as a function of the delayτin the Michelson setup ofFigure 2b. (a) Experimentalg(2)features (black) of degenerate twin beams compared with quantum modelling (magenta) and chaotic light with the same spectrum (experimental in olive and modelling in green). The inset shows the twin-beam spectrum at degeneracy. (b) Experimentalg(2)features (black) of twin beams far from degeneracy compared with modelling expectation (magenta) and chaotic light with the same spectrum (green) (equivalent to two independent chaotic sources presenting, respectively, the same signal spectrum and idler spectrum). The inset shows the twin-beam spectrum far from degeneracy. Blue line is named signal radiation and red line idler radiation. Figure 4a and b are, respectively, related to the spectrum shown in the insets, that is, very close to degeneracy ( Fig. 4a ; λ s , i =1.56 μm) and far from degeneracy ( Fig. 4b ; λ s =1.4 μm and λ i =1.7 μm). The same experiments are realized on incoherent light beams (olive curves), for example, obtained by tuning out the dispersion compensation setup [30] . All g (2) experimental curves are compared with the result of a full quantum calculation presented in ref. 30 (Methods) and with what would be obtained with uncorrelated chaotic sources (for example, ref. 7 ). Both at degeneracy and far from degeneracy, the measured value of the second-order coherence function at zero time delay is g (2) (0)≈3±0.15, whereas values obtained with chaotic sources are, as is well known, This striking 'extrabunching' effect, also referred as enhanced photon bunching, has been theoretically predicted, for example, in refs 7 , 28 . Away from degeneracy, one observes an additional modulation of g (2) ( τ ), occurring at the beat frequency ω s − ω i (refs 30 , 39 ). Figure 4: Quantitative measurements of extrabunching. g (2) ( τ ) as a function of the delay τ in the Michelson setup of Figure 2b . ( a ) Experimental g (2) features (black) of degenerate twin beams compared with quantum modelling (magenta) and chaotic light with the same spectrum (experimental in olive and modelling in green). The inset shows the twin-beam spectrum at degeneracy. ( b ) Experimental g (2) features (black) of twin beams far from degeneracy compared with modelling expectation (magenta) and chaotic light with the same spectrum (green) (equivalent to two independent chaotic sources presenting, respectively, the same signal spectrum and idler spectrum). The inset shows the twin-beam spectrum far from degeneracy. Blue line is named signal radiation and red line idler radiation. Full size image Such oscillations are inexistent in the modified Mach–Zehnder setup ( Fig. 2c ) as only one path is possible for coincident signal–idler photons in this experiment. 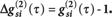Figure 5: Cross-correlation function This curve is obtained by using the modified Mach–Zehnder apparatus ofFigure 2c. Experimental cross-correlation function of twin beams far from degeneracy (black) is compared with quantum modelling (magenta) and chaotic light (green) with the same spectrum. The orange dashed curve is the twin-beam cross-correlation functionderived from data inFigure 4b. Figure 5 shows the additional (see equation (5)) extracted from TPC MZ ( τ ) as a function of the time delay τ between signal and idler (Methods). As in the Michelson configuration, we observe an unambiguous extrabunching effect compared with the chaotic sources [7] , with a value 1±0.2 instead of 0 for uncorrelated sources. The magenta curve is the result of quantum modelling with no fitting parameter [30] (Methods). Figure 5: Cross-correlation function This curve is obtained by using the modified Mach–Zehnder apparatus of Figure 2c . Experimental cross-correlation function of twin beams far from degeneracy (black) is compared with quantum modelling (magenta) and chaotic light (green) with the same spectrum. The orange dashed curve is the twin-beam cross-correlation function derived from data in Figure 4b . Full size image To describe our experimental results and explain the extrabunching effect, we can first use a simple quantum model: The quantum state describing a pulse of down-converted light is [40] : with equal photon numbers in the signal and idler modes ( n s = n i = n ), supposed here to be monochromatic in a first simple approach, G being the intensity parametric gain in the non-linear crystal. Using this expression, one can easily calculate the correlation functions at zero time delay. One obtains: In our experiment, the parametric gain G is roughly 2.5×10 7 , so that one gets the limit values 3 for g (2) (0) and 1 for in agreement with the experimental data. As these approaches do not allow to track intuitively the physical origin of the extrabunching effect, we need to have a closer look at the TPA process and how it is involved in the two different experimental setups. Let us use, as an educated guess, a semiclassical description of the SPDC field, inspired by the atomic radiation model of ref. 7 . The signal or idler field separately considered are expressed as a sum over a large number ν of independent radiating dipoles ( ν ≫ 1) at a mean frequency ω k as where E k 0 is the dipole amplitude and ϕ k , j ( t ) is the phase angle for the field ' k ' from the ' j ' dipole [7] . Phases ϕ k , j ( t ) for different ' j ' dipoles (but same ' k ' field) are completely unrelated, thus exhibiting the usual chaotic behaviour [7] , [35] . Nevertheless, for the same ' j ' dipole, one has the following relation on the sum of signal and idler phases: This relation can be derived from the semiclassical equations of parametric interaction [40] . Using equations (8) and (9), equation (2) can be rewritten as where Equation (10) enlightens the origin of the signal–idler cross-correlation. The first term (that is, 1) originates from accidental coincidences between photons of the two uncorrelated sources while the second one stems from exact coincidences between twin photons (that is, This last term is zero in the case of uncorrelated chaotic sources. Consequently, the Mach–Zehnder setup is a direct measurement of these exact coincidence correlation terms. Moreover, being the signal–idler field cross-correlation, one can easily understand the dependence of the measured extrabunching magnitude on the chromatic dispersion. The Michelson setup yields more complex but richer physical parameters on the second-order coherence of the SPDC light as it measures the g (2) ( τ ) function of the total field (including g (2) (0)=3). Without going further into the mathematical development, the last terms of equation (3) can be related to usual first-order correlation function by: where only main contributions of a large number of radiating dipoles were kept and the modulation component was intentionally emphasized. In equation (11), the first term in curly brackets is related to the superposition of signal and idler single beam interferences, whereas the second one results from additional twin-beam phase relation described in equation (9). One thus recovers the oscillations at the beating frequency ω s − ω i observed in Figure 4b for twin beams and chaotic light. Using equations (3) and (11), one can extract the cross-correlation term from the experimental data in Figure 4 (Michelson data), which is compared in Figure 5 (orange dashed curve) with the one extracted from the Mach–Zehnder experiment (black curve). Both curves are in excellent agreement. The twin-beam coherence time determined from the curves (both theoretical and experimental) ranges from 65±3 fs (degeneracy) to about 245±30 fs (far from degeneracy; Figs 4 and 5 ). They are linked to the spectral acceptance of the parametric processes and are in excellent agreement with theoretical expectations (Methods). In conclusion, owing to the huge bandwidth offered by the TPC experiments, the long searched photon extrabunching effect in twin beams has been observed and quantitatively measured. In agreement with theoretical calculations, the specific twin-beam correlation properties lead to a striking enhancement of g (2) , g (2) (0)=3 for a high photon flux, when compared with chaotic light with the same spectrum. These results firmly establish TPC in semiconductors as a powerful tool for the absolute measurement of light beam photon correlations at ultrashort timescales. Physical insights on the origin of the extrabunching effect have been gained by use of a semiclassical description of SPDC light as a sum of uncorrelated 'twin dipoles'. Finally, TPC apparatus allows the unique possibility of measuring the coherence properties of two light beams with an extremely large gap in frequencies. This will open new routes in the fields of Lidar and non-linear spectroscopy. Data normalization procedure for Michelson setup As shown in ref. 29 , a proper normalization of TPC LPF ( τ ), which is obtained after a numeric low-pass filtering of the interferogram, enables to directly derive the function g (2) ( τ ): where τ c is the photon correlation time whose order of magnitude is around 100 fs in our case. We typically chose τ ≈500 fs to carry out the normalization procedure in order to remain much shorter than the pump pulse duration. The increase of g (2) (0) for twin beams when compared with incoherent light is directly observable on the raw data of Figure 3 from the fact that the shoulders of TPC LPF ( τ ) around the narrow central peak (red curve in Fig. 2a ) are at 5/3 (twin beams) instead of 2 (incoherent light). Data normalization procedure for Mach–Zehnder setup In an analogous way as for the Michelson interferometer, can be derived from raw data after a simpler normalization procedure. The initial twin beams are split apart by a dichroic mirror in a signal beam and an idler beam, which are recombined (with a variable delay on the signal path) on the two-photon detector ( Fig. 2c ). Thus, in a continuous-mode quantum approach, the TPC response is proportional to: where is the creation field operator related to the 'idler' ('signal') path, thus reduced to the idler (signal) frequency domain, that is, 0< ω < ω p /2 ( ω p /2< ω < ω p ). Divided by the sum of mean TPC from each path, that is, the normalized TPC rate can be expressed easily as: The cross-correlation is thus given by: Determination of correlation times Calculations of correlation time are based on a Gaussian approximation [7] , that is, first-order correlation functions are given by: where is the field correlation time (well-known coherence time for k = l ). Modelling parameters According to the modelling briefly developed in ref. 30 , we suppose here that dispersion phenomena are well compensated and there is no loss. Twin-beam state at the detector is thus given by the one at the exit of the PPLN non-linear crystal. Very few parameters are needed and can all be measured. We determined and used the following parameters in the present paper modelling: Non-linear crystal: length 35 mm; effective non-linear coefficient d eff =16 pm V −1 ; quasi-phase matching period 18.9 μm; and temperature 125.5 °C (degeneracy) 136.3 °C (far from degeneracy). Pump parameter: wavelength 780 nm; beam diameter in the non-linear crystal is about 120 μm; mean pump power 2 W; and modelling was carried out using a continuous pump at peak pump power calculated from mean pump power, laser pulse duration and repetition rate. How to cite this article: Boitier, F. et al . Photon extrabunching of ultrabright twin beams measured by two-photon counting in a semiconductor. Nat. Commun. 2:425 doi: 10.1038/ncomms 1423 (2011).